Ranking stability and super-stable nodes in complex networks Pagerank, a network-based diffusion algorithm, has emerged as the leading method to rank web content, ecological species and even scientists. Despite its wide use, it remains unknown how the structure of the network on which it operates affects its performance. Here we show that for random networks the ranking provided by pagerank is sensitive to perturbations in the network topology, making it unreliable for incomplete or noisy systems. In contrast, in scale-free networks we predict analytically the emergence of super-stable nodes whose ranking is exceptionally stable to perturbations. We calculate the dependence of the number of super-stable nodes on network characteristics and demonstrate their presence in real networks, in agreement with the analytical predictions. These results not only deepen our understanding of the interplay between network topology and dynamical processes but also have implications in all areas where ranking has a role, from science to marketing. Originally introduced to rank web pages in the world wide web (www) [1] , pagerank, a network-based diffusion algorithm, today is not only at the heart of Google and other search engines [2] but also the method of choice for ranking an extensive array of data in a wide range of network environments. It is used to rank physicists based on their citation patterns [3] , [4] , disease-causing genes based on protein–protein interactions [5] , academic doctoral programs based on alumni placement [6] , roads or streets in terms of traffic [7] , ecological species based on their position in the food web [8] , highlight cancer genes in proteomic data [9] and even to disambiguate words in lexical semantics [10] . The algorithm's popularity lies in both its perceived effectiveness and its easy to understand philosophy: rather than ranking objects based on difficult-to-measure intrinsic qualities, such as the utility of a webpage or the creativity of a researcher, it exploits the collective wisdom encoded in the network the object is part of, interpreting each link as an inherent vote. Current advances in the statistical mechanics of complex networks [11] , [12] , [13] , [14] , [15] , [16] , [17] , [18] have shown that the systems on which pagerank operates have significant differences in their network topology: some, such as the www, are scale-free [19] , [20] , others, such as food webs, display a mixture of exponential and fat-tailed degree distributions [21] ; the underlying networks have different sizes, average degree, path length, degree correlations [22] , [23] and community decomposition [24] , [25] , [26] . These topological differences are known to affect most network-based processes, from epidemic spreading [27] , [28] to diffusion and network robustness [29] , [30] , [31] , [32] , [33] , [34] . Yet the role of the underlying network structure in the effectiveness of pagerank remains unknown, prompting us to ask: could pagerank be inherently more accurate for some networks than for others? The key role ranking has from information retrieval to marketing makes this a question of major practical importance, affecting many aspects of our information society [35] . Although the stability of pagerank to perturbations has been studied in computer science [36] , [37] , [38] , [39] , we will show here that by focusing on the ranking stability of the top nodes we can obtain a series of fundamental results, that reshape our understanding of ranking stability. In particular, we find that, thanks to the fat-tailed nature of the degree distribution, a few super-stable nodes can emerge whose ranking becomes independent of what other nodes connect to them. We demonstrate the presence of such super-stable nodes in several real systems, from the www to citation networks. Pagerank algorithm and diffusion The pagerank of a node in a network of N nodes with adjacency matrix A ij can be calculated from where k out ( j ) is the number of outgoing links from node j and α is a reset parameter [1] . Equation (1) describes a diffusion process, where p t ( i ) is the frequency of visitation of node i by a particle at time step t that moves along the links of the network (encoded in the adjacency matrix A ij ) with probability α and jumps to a randomly chosen node with probability 1− α . The stationary state of this diffusion process is the pagerank p ( i ) of node i , determining its ranking relative to other nodes. In addition to its link to diffusion, mapping equation (1) to a Schrödinger-like wave equation helps elucidate the localization properties of the web graph [40] , [41] . The central hypothesis of the pagerank algorithm is that a link from a node i to node j serves as an 'endorsement' of node j by i . Moreover, the status of the recommending node is important—a letter of recommendation from a Nobel Laureate (that is, a node with high pagerank p t −1 ( j )) carries far more weight than 10 letters from academics of lesser prominence. However, if the Laureate has drafted a large number of recommendations for various candidates (has a high k out ( j )), then his (her) status as a recommender drops. Pagerank typically operates on networks that are either mapped incompletely, such as the www [42] , or contain many false positives and negatives, such as protein interaction networks [43] , raising a fundamental question: is the ranking of a node stable relative to other nodes in the face of such considerable network perturbations? Ranking stability under degree-preserving perturbations As random perturbations, from network incompleteness to noise, leave the relative degrees of the nodes largely unaltered, here we study the ranking stability under degree-preserving perturbations. This is achieved by randomly rewiring the network, while leaving the degree of each node (and hence the degree distribution P ( k )) invariant. This approach is also motivated by the fact that the leading contribution to the pagerank of a node is its in-degree [44] , therefore perturbations that randomly change a node's degree render the algorithm useless. The ranking of a node with rank m is considered stable under network perturbations if changes in its pagerank p m (where the subscript associates the pagerank to its rank, that is, the node with the highest pagerank has m =1) leave the node's ranking m unchanged. Denoting with σ ( p m ) the fluctuations in p m around its mean value 〈 p m 〉 under different realizations of the degree-preserving perturbations, the m th ranked node has a stable rank if where Δ( p m )= p m − p m +1 . In other words, if the fluctuations in a node's pagerank p m are small compared with the gap between its pagerank p m and that of the node ranked below it p m +1 , the perturbation will not lower its ranking. Note, that Δ( p m )/ σ ( p m ) is a monotonically decreasing function in m ; hence, if the gap exceeds the fluctuation for a specific rank m , then it will also exceed for all m ′< m . To see whether the stability criteria equation (2) is ever satisfied, we calculated analytically the expected gap and fluctuations in the pagerank for networks with different degree distributions ( Supplementary Methods , Supplementary Figs S1 and S2 ). We find that for a scale-free network ( P SF ( k ) ∼ k − γ ) [19] , the gap follows , whereas for an exponential network ( P exp ( k ) ∼ e − λ k ) [45] , we have . The fluctuations σ ( p m ) in scale-free networks follow , whereas in exponential networks . Therefore, the stability ratio for the two networks is where the complete expressions for F SF and F exp are provided in Supplementary Methods . Note that although the stability ratio equation (3) for scale-free networks depends on the system size, N , for exponential networks equation (4) is size invariant. The reason is that for an exponential distribution the top nodes have comparable degrees ( Fig. 1a ), whereas for a fat-tailed distribution ( Fig. 1b ) the degrees of the top nodes are well separated from each other. Indeed, the relative gap, ( k max − k max−1 )/ k max−1 between the two top-ranked nodes in exponential networks of size N =10 4 is ∼ 10 −2 ( Fig. 1c ), whereas for scale-free networks it is 10 0 −10 1 , that is, two–three orders of magnitude larger ( Fig. 1d ). Consequently in an exponential network, the pagerank distribution of the top nodes are practically indistinguishable ( Fig. 1e ), indicating that the identity of the first-, second- or third-ranked node is different for each configuration. In contrast, the pagerank of the top node is well separated from the pagerank of the second- and third-ranked nodes in a scale-free network ( Fig. 1f ), indicating that the top-ranked node remains the same for each network configuration, being insensitive to perturbations. 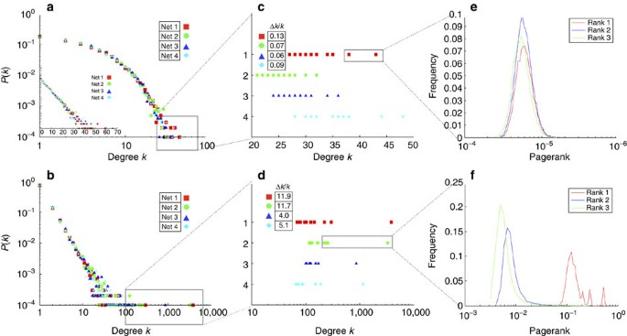Figure 1: The difference between exponential and scale-free distributions. The degree distributions of (a) four networks with exponential degree distributionP(k)∼e−λkwithλ=0.2 on a log–log scale (inset: log-linear) and (b) four networks with scale-free degree distributionP(k)∼k−γwithγ=2.2, average degree 〈k〉=5 and sizeN=104. (c,d) The magnified area of a and b showing the gap between the largest degrees. The difference between the largest degrees in a scale-free network is consistently large compared with the largest values in an exponential network. The legend shows the relative difference in the top two degrees' Δk=(kmax−kmax−1)/kmax−1) for both degree distributions. (e,f) The pagerank distributions of the top three nodes selected from each network type. For the power law distribution, the peak of each curve can be clearly distinguished in contrast with the exponential network where the top nodes' pagerank are practically indistinguishable. Figure 1: The difference between exponential and scale-free distributions. The degree distributions of ( a ) four networks with exponential degree distribution P ( k ) ∼ e − λ k with λ =0.2 on a log–log scale (inset: log-linear) and ( b ) four networks with scale-free degree distribution P ( k ) ∼ k − γ with γ =2.2, average degree 〈 k 〉=5 and size N =10 4 . ( c , d ) The magnified area of a and b showing the gap between the largest degrees. The difference between the largest degrees in a scale-free network is consistently large compared with the largest values in an exponential network. The legend shows the relative difference in the top two degrees' Δ k =( k max − k max−1 )/ k max−1 ) for both degree distributions. ( e , f ) The pagerank distributions of the top three nodes selected from each network type. For the power law distribution, the peak of each curve can be clearly distinguished in contrast with the exponential network where the top nodes' pagerank are practically indistinguishable. Full size image Equation (4) predicts that for an exponential network the gap between consecutive pageranks never exceeds the fluctuations, making the ranking rather sensitive to perturbations. In contrast, according to equation (3), for certain ( N , γ and α ) combinations in a scale-free network the stability criteria equation (2) is satisfied, predicting the existence of a finite set of nodes whose ranking is stable to network perturbations. We will call these nodes super-stable, which means that by virtue of the many links they have, their ranking is independent of who points at them. Thus, degree-preserving perturbations do not alter their ranking, in contrast with the rest of the nodes in the network, whose ranking is sensitive to precisely which node points at them. 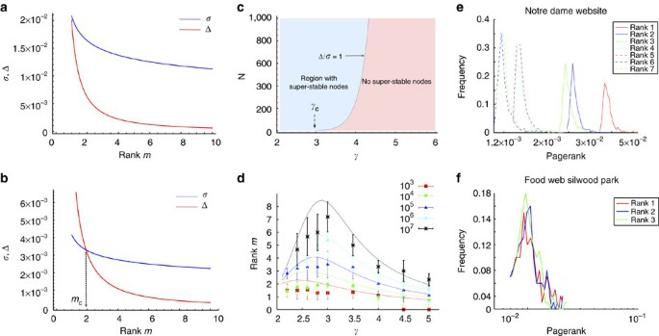Figure 2: Analytical and numerical evidence for super-stable nodes. (a,b) Pagerank gap Δ(pm) and the fluctuationσ(pm) plotted as function of the rankmfor two scale-free networks with the same exponent,γ=3.5, and different system sizes,N=102and 104¸ showing the emergence of super-stability for largerN. (c) The (N,γ) phase diagram showing the stable and unstable regimes that emerge forγ>γc=3. (d) The critical rankmcas a function ofγwhere the curves correspond to the calculatedmcand the points represent the measuredmcin numerical simulations on multiple networks. The peak nearγc=3 is more pronounced asNincreases, with different scaling behaviors above and belowγc. (e,f) Pagerank distributions of the top-ranked nodes in the www (scale-free) and the food web (exponential) shown inTable 1. The separated curves correspond tomc(measured) values shown in the table. Note that in the www the top-ranked nodes are clearly identifiable, whereas in the food web there are no super-stable nodes as predicted by the calculation. In Figure 2a,b, we show Δ( p m ) and σ ( p m ) for the top-ranked nodes in scale-free networks with sizes N =10 2 and 10 4 . For N =10 2 , the fluctuations σ exceed the gap Δ for any rank m , indicating the absence of nodes whose rank is stable to perturbations. However, for N =10 4 nodes with m < m c , we have σ ( p m )<Δ( p m ), indicating that their rank is stable. In general, the stability ratio Δ( p m )/ σ ( p m ) scales with system size as N 1 / 2 ( γ - 1 ) (a dependence absent in exponential networks), that is, the larger the scale-free network the more stable is the ranking of the top nodes. Therefore, it is easier to agree on the relative ranking of the top nodes in a large network than a small one, a rather counterintuitive result, given the cognitive limits that we face when we try to compare with each other a larger number of objects or services. The reason is that in larger systems the likelihood of the emergence of true outliers, whose pagerank is significantly greater than others, is greater. Figure 2: Analytical and numerical evidence for super-stable nodes. ( a , b ) Pagerank gap Δ( p m ) and the fluctuation σ ( p m ) plotted as function of the rank m for two scale-free networks with the same exponent, γ =3.5, and different system sizes, N =10 2 and 10 4 ¸ showing the emergence of super-stability for larger N . ( c ) The ( N , γ ) phase diagram showing the stable and unstable regimes that emerge for γ > γ c =3. ( d ) The critical rank m c as a function of γ where the curves correspond to the calculated m c and the points represent the measured m c in numerical simulations on multiple networks. The peak near γ c =3 is more pronounced as N increases, with different scaling behaviors above and below γ c . ( e , f ) Pagerank distributions of the top-ranked nodes in the www (scale-free) and the food web (exponential) shown in Table 1 . The separated curves correspond to m c (measured) values shown in the table. Note that in the www the top-ranked nodes are clearly identifiable, whereas in the food web there are no super-stable nodes as predicted by the calculation. Full size image Figure 2a,b suggests that the system size must exceed a critical size for super-stable nodes to emerge. Defining N c as the minimum system size for which at least the top node's ranking is stable (that is, Δ( p 1 )/ σ ( p 1 )≥1), we find that for scale-free networks with degree exponents in the range 2≤ γ <3 we have N c =0, indicating that super-stable nodes emerge for any system size. For γ ≥3, however, only networks whose size exceeds can have super-stable nodes ( Supplementary Methods ). Therefore, γ c =3 represents a critical exponent for ranking stability, as illustrated by the ( N , γ ) phase diagram of Figure 2c : for γ < γ c =3, we always have at least one super-stable node, whereas for γ > γ c only for N > N c ( γ ) can super-stability emerge. We also find that the number of super-stable nodes m c scales as m c ∼ N 1/(2 γ −1) , which is a rather weak dependence—for γ =3, to increase m c by a factor of ten, one needs to increase the system size by five orders of magnitude. For large N and 2< γ <3, the critical rank m c depends on γ as e A( γ −2)/(2 γ −1) and for γ ≫ 3, it decays as γ − γ . The resulting γ dependence is summarized in Figure 2d , indicating that the number of stable ranks is relatively small for all γ and that it peaks in the vicinity of γ c =3. The peak becomes increasingly pronounced for large N . At the first glance, the peak at γ c =3 is unexpected: an increasing γ should decrease the gap as Δ( p m ) ∼ N 1/2( γ −1) . Note, however, that for γ <3 the fluctuations σ ( p m ) diverge as σ ∼ N (3− γ )/( γ −1) , whereas σ ( p m ) is asymptotically size independent for γ >3. Hence for γ <3, the gap is large but so are the fluctuations, whereas for γ >3 the gap decreases and the fluctuations are effectively constant. The best payoff between these two regimes is in the vicinity of γ c =3, where σ 2 ∼ (1/2)log( N π ), resulting in the peak at γ c ( Supplementary Methods ). To test our analytical predictions, we generated networks with fixed P ( k ) using the configuration model [46] , and then ranked each node according to their pagerank. We perturbed the network by rewiring every edge (keeping the degree of each node unchanged) and determined the pagerank after each rewiring, helping us identify nodes whose ranking did not change as a result of the perturbation. We not only found that such nodes exist in the predicted topological regimes, but also plot the measured value of the critical rank m c as a function of the exponent γ for various system sizes in Figure 2d , confirming the predicted trend: for large N , the m c versus γ curves develop a peak in the vicinity of γ c . Most importantly, the analytical and the numerical results agree that the number of super-stable nodes is rather small—less than ten for a system with ten million nodes. Evidence of super-stable nodes in real networks To see whether super-stable nodes emerge in real systems, we collected data for a variety of real networks, ranging from samples of the www to citation networks and identified the nodes whose ranking do not change under rewiring perturbations. For each network with a fat-tailed degree distribution, we observed a few super-stable nodes whose number closely agrees with the analytical prediction ( Table 1 ). For networks with an exponential degree distribution, the data support our prediction that super-stable nodes are absent. The only exception is the neural network of Caenorhabditis elegans , which has one super-stable node, because of the fact that its in-degree is separated by an order of magnitude from the rest of the nodes. Note that the probability to have such a high in-degree in this network is ∼ 10 −9 , indicating that this node, a motor neuron responsible for locomotion, represents a clear deviation from the expected degree distribution. The different behavior of the pagerank for the two network classes is illustrated in Figure 2e,f , where we show the pagerank distributions for the top nodes in two networks, the www (scale-free) and the food web (exponential). In line with our predictions, for the www, the top nodes are clearly separated from the rest of the nodes, whereas for the food web the pagerank distributions of the top nodes are indistinguishable. Table 1 Super-stable nodes in real networks. Full size table Probably, the strongest direct evidence supporting our predictions comes from the Physical Review citation network. We used the publication history of papers published in the Physical Review journals from 1893 to 2009, allowing us not only to identify the super-stable nodes from a static snapshot of the citation network, but also to track the emergence of super-stability in time. Two systematic changes in the network impact the number of super-stable nodes: (i) The network grows, increasing from N =0 in 1892 to N =449,673 in 2009 ( Fig. 3a ). (ii) The degree exponent decreases from γ ≈5 in the 1950s to γ ≈3 today ( Supplementary Fig. S3 ). We therefore predicted the number of super-stable nodes in each decade between 1900 and 2000, by incorporating the changes in N and γ , and also identified m c directly from the real data. We find that super-stable papers do not emerge before the 1950s, as the combination of high-degree exponent and small N prohibits super-stability ( Fig. 3b ). However, as the degree exponent γ drops and N increases, between 1950 and 1960, N overcomes N c , allowing for the emergence of the first super-stable paper ( m c =1). In the subsequent decades, m c gradually increases to four super-stable papers. 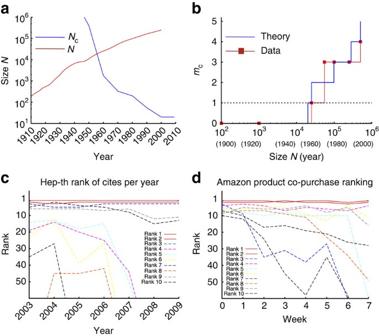Figure 3: Temporal stability of super-stable nodes. (a) The number of papers published in the Physical Review corpus with time and the predicted critical system sizeNc. (b) The evolution of the number of super-stable nodes in the same network,mc, as a function of size,N, and time (shown in parentheses). The squares correspond to the measuredmcfrom the Physical Review citation network, whereas the curve corresponds to the analytical prediction using the appropriateNand the best estimate ofγfor each decade. (c) The number of citations per year for the top ten ranked papers, where ranking is provided by applying pagerank to all high-energy physics papers published by 2002. The two predicted super-stable nodes (solid red lines) continue to be the top cited papers for almost a decade. The rest of the papers display considerable fluctuations in rank, even dropping out of the top 50 lists. (d) The evolution of the ranks of the top ten most co-purchased books in Amazon. The curves represent the evolution of books, ranked in the top ten in our first sample, over the subsequent weeks. Although the ranking of most nodes fluctuate, the top two nodes—predicted to be super-stable (solid red lines)—maintain their top ranking. As Figure 3b shows, the numerically identified m c closely follows the analytical predictions, the difference being at most one super-stable paper in a decade. Hence, the data set not only confirms the existence of super-stable publications in the Physical Review corpus (for the list of super-stable papers, see Supplementary Table S1 ), but also shows that their emergence in time follows closely the analytical predictions. Figure 3: Temporal stability of super-stable nodes. ( a ) The number of papers published in the Physical Review corpus with time and the predicted critical system size N c . ( b ) The evolution of the number of super-stable nodes in the same network, m c , as a function of size, N , and time (shown in parentheses). The squares correspond to the measured m c from the Physical Review citation network, whereas the curve corresponds to the analytical prediction using the appropriate N and the best estimate of γ for each decade. ( c ) The number of citations per year for the top ten ranked papers, where ranking is provided by applying pagerank to all high-energy physics papers published by 2002. The two predicted super-stable nodes (solid red lines) continue to be the top cited papers for almost a decade. The rest of the papers display considerable fluctuations in rank, even dropping out of the top 50 lists. ( d ) The evolution of the ranks of the top ten most co-purchased books in Amazon. The curves represent the evolution of books, ranked in the top ten in our first sample, over the subsequent weeks. Although the ranking of most nodes fluctuate, the top two nodes—predicted to be super-stable (solid red lines)—maintain their top ranking. Full size image Our ability to identify super-stable nodes from a single snapshot of the network raises an important question: how stable is the ranking with time? To answer this question, we collected time-resolved ranking data for the citation and co-purchasing networks ( Supplementary Table S2 ), allowing us to quantify the temporal stability of the top nodes. In the high-energy citation network, the super-stable nodes were identified from a sample containing all papers published in 2002. We find, however, that in the subsequent 7 years these two papers maintain their top ranking, collecting the most citations each year. In contrast, the ranking of the rest of the papers, which do not demonstrate super-stability in the 2002 sample, fluctuates widely ( Fig. 3c ). Similarly, for the Amazon co-purchasing network, the two super-stable books continue to maintain their rank in samples collected on a weekly basis ( Fig. 3d ) and were the top ranked in a sample collected 6 years earlier (2005) as well. Additionally, in the Physical Review Corpus ( Supplementary Fig. S4 ), most super-stable nodes maintain their status for a period of 6–10 years; some, such as the 1957 paper on the BCS theory of superconductivity, show super-stability for three decades. Taken together, we find that super-stable nodes, identified from a single snapshot of the network, show a remarkable temporal stability, a feature not shared by other nodes in the system. In summary, we find that real networks with heavy-tailed degree distributions naturally lead to a set of super-stable nodes that have such a high number of 'recommendations' (in-degree) that their ranking becomes independent of who recommends them. This is somewhat unexpected from the perspective of the network architecture: the scale-free nature of these networks normally implies a lack of objective criteria to distinguish hubs from non-hubs. The balance of rank stability and fluctuations do allow us, however, to identify a few hubs that respond in a distinct manner to perturbations. Both our analytical predictions and numerical results indicate that the number of super-stable nodes is very small. As predicted by our scaling analysis, this number is largely unaffected by most network characteristics and only a significant increase in system size can increase their number. This suggests that across a large number of systems a small number of components (nodes) are bound to have a disproportionate role in the system. These nodes are often easy to identify: a simple link counting should place them at the top, limiting the usefulness of pagerank to rank nodes that are not super-stable. It is often mentioned that the early success of Google compared with its competitors was not because of better coverage (which back then was inferior to that of the market leader Inktomi), but its pagerank algorithm, that offered a superior user experience through a better ranking of the relevant documents. Our results suggest that the success of pagerank was the inadvertent consequence of the scale-free nature of the web graph. Had the web been an exponential network, the ranking provided by pagerank would have been unreliable given the incompleteness of the web graph. Indeed, in 1999, Google indexed only 7.8% of the web [42] and even today its coverage is less than half of the indexable web. Yet, the scale-free property of the web graph leads to the emergence of a small number of super-stable nodes, for which a simple count of the in-degree offers the correct relative ranking. As the www grew, the ranking stability at the top increased, making the top-ranked nodes even easier to identify. Therefore, counterintuitively, we find that the growth of the web, instead of making search more difficult by offering more hits, helps select clear winners, offering better ranking clarity at the top. Determining the gap and fluctuation in pagerank Given a probability distribution p ( x ), we can determine the expectation value of the largest x after we draw N numbers from p ( x ). If we draw N numbers from a particular sample and one of them, x i , lies between the interval x +d x , the probability that there are no other numbers with a greater value than x i is given by p ( x )d x ×[1− P ( x )] N −1 , where P ( x ) is the cumulative distribution. As there are N ways of choosing x i , the total probability is π ( x )= Np ( x )(1− P ( x )) N −1 . Similarly, we can determine the expectation value of the m th largest number 〈 x 〉 m . By definition, the m th ranked number has m −1 numbers above it and N − m below it, obtaining where the denominator is the beta function. The expectation value is determined by, Combining this with equation S1 ( Supplementary Methods ) gives the expectation value for the pagerank p m of a node ranked m . The gap between the pagerank of a node ranked m and the node ranked one place below it p m +1 is Δ( p m )= p m − p m +1 , whereas the fluctuation σ ( p m ) is determined by substituting p m into equation S2 . The details of the calculation are listed in Supplementary Methods . Determination of critical values According to the stability criteria equation (2), setting the ratio Δ( p m )/ σ ( p m ) equal to one allows us to define a critical value for each relevant parameter, such that above that value we are in the stable regime and below in the unstable regime. We focus on two parameters: the critical system size N = N c , which specifies the minimum system size for which any stable ranks exist, and m = m c , which denotes the maximum rank in the network that is stable for system size N > N c . To find N c in a scale-free network, we note that the maximum value of equation (3) as a function of m is at m =1. Furthermore, the ratio is a monotonically decreasing function in m ; hence, if there is a critical value for the system size N c , then it must at least hold for m =1 and thus setting the ratio and m equal to one, we can derive an equation for N c . The equation can only be solved numerically, but the scaling behavior of N c can be extracted through a series of approximations ( Supplementary Methods ). Similarly, the critical rank m c is derived by setting the ratio to one and N to a fixed value N > N c . How to cite this article: Ghoshal, G. & Barabási, A.-L. Ranking stability and super-stable nodes in complex networks. Nat. Commun. 2:394 doi: 10.1038/ncomms1396 (2011).